A drug-specific nanocarrier design for efficient anticancer therapy The drug-loading properties of nanocarriers depend on the chemical structures and properties of their building blocks. Here we customize telodendrimers (linear dendritic copolymer) to design a nanocarrier with improved in vivo drug delivery characteristics. We do a virtual screen of a library of small molecules to identify the optimal building blocks for precise telodendrimer synthesis using peptide chemistry. With rationally designed telodendrimer architectures, we then optimize the drug-binding affinity of a nanocarrier by introducing an optimal drug-binding molecule (DBM) without sacrificing the stability of the nanocarrier. To validate the computational predictions, we synthesize a series of nanocarriers and evaluate systematically for doxorubicin delivery. Rhein-containing nanocarriers have sustained drug release, prolonged circulation, increased tolerated dose, reduced toxicity, effective tumour targeting and superior anticancer effects owing to favourable doxorubicin-binding affinity and improved nanoparticle stability. This study demonstrates the feasibility and versatility of the de novo design of telodendrimer nanocarriers for specific drug molecules, which is a promising approach to transform nanocarrier development for drug delivery. Nanoparticle-based drug encapsulation increases drug solubility and stability, minimizes toxic side effects [1] , [2] and, more importantly, delivers drug molecules specifically to tumours through the enhanced permeability and retention (EPR) effect [3] , [4] . Several nanodrugs have been approved by US Food and Drug Administration [1] , [5] . For example, Doxil, a stealth liposomal nanoformulation of doxorubicin (DOX), has significantly reduced cardiotoxicity [6] . However, Doxil shows only marginal improvement in efficacy over free DOX in clinical practice, especially for solid tumour treatment [6] , [7] , [8] . It is because of the poor intratumoral diffusion ( ∼ 100 nm) (ref. 7 ) and unfavourable drug release profile reducing drug availability, despite more drug delivered to tumour sites by EPR effects [6] , [7] , [8] . This indicates that the balance between drug retention and drug release is critical in determining the in vivo fate and efficacy of a nanoformulation in cancer treatment. In the literatures, numerous DOX delivery systems have been developed including liposomes [9] , dendrimers [10] , [11] , polymer nanoparticles [12] , polymer–DOX conjugations [13] , [14] , polymer micelles [15] , [16] and inorganic nanoparticles [17] . Of these, polymer micelles (10–100 nm in size) are one of the most versatile nanocarriers for the delivery of DOX and other chemotherapeutic drugs because of the abundant chemical diversity, functionality and tunable physical properties [16] . ‘Like dissolves like’ is a principle rule that is applicable to mixture systems. A docetaxel-conjugated polyethylene glycol-poly(ɛ-caprolactone) (PEG-PCL) polymer showed higher docetaxel-loading capacity and stability than the parent polymer PEG-PCL [18] . Polymer–drug conjugations via labile bonds are considered to be an effective prodrug strategy to increase the solubility and reduce the toxicity of the hydrophobic drug molecules [14] , [19] . Despite the fact that some polymeric prodrugs can self-assemble into micelles for further drug loading [18] , this approach may be hindered by the availability of functional groups on a drug molecule and the high cost of production. Instead, a molecule with structural similarity and a complimentary conformation to the drug molecule is promising as an efficient host after being conjugated on a polymeric nanocarrier to improve drug delivery. However, it is still challenging to introduce these molecules freely into polymers with the precise control of location and density. The growth of the polymer field has benefited from new developments in synthetic and catalytic chemistry. The biocompatible polymers for drug delivery are still limited to a few, which hinders the development and optimization of nanocarriers to deliver the compounds/drugs in preclinical and clinical development. In addition, the uncertain relationship between the structure and property of polymer nanoparticles for drug delivery is a problem for pharmaceutical companies, whose expertise is to probe the well-defined drug–biologic interactions using systematic and computer-aided approaches [20] . Computational chemistries, such as theoretical methods and molecular simulations, have been applied in nanoparticle system to understand drug-loading properties [21] . Unlike proteins, nanoparticle systems have no defined conformations and are too big in size for computation chemistry to build an affordable and reliable model for drug-loading predictions. Up-to-date, the structure-based de novo design and optimization of nanocarriers for a given drug delivery has not been documented because of the lack of both reliable theoretical models and precise polymer synthesis for the systematic validation and evaluation [21] . Here we developed a novel well-defined telodendrimer nanoplatform to leverage the synergism between computational design and combinatorial chemistry for drug-specific nanocarrier development. We found that the optimized telodendrimer nanoformulations of DOX significantly improved the treatment of lymphoma in animal models, in comparison with free DOX and Doxil. A well-defined nanoplatform We have developed a hybrid polymer system, a telodendrimer, composed of linear polyethylene glycol (PEG)-blocking-dendritic polylysine and the capping peripheral building blocks, for example, cholic acid (CA) [22] , [23] . It self-assembles into micelles in aqueous solution for efficient delivery of anticancer drugs [22] , [23] , [24] , [25] , [26] , [27] , [28] . The efficient peptide chemistry used in telodendrimer synthesis allows for free and precise control over the architecture and the functionality of the telodendrimer. The peripheral groups on the dendritic polylysine have more flexibility in interacting with drug molecules when compared with the main chains or pendant groups in linear polymers. This interaction greatly influences drug-loading properties of nanocarriers. We hypothesize that the optimal drug-binding molecules (DBMs) could be identified by molecular docking and introduced into telodendrimer in parallel to make a library of nanocarriers for systematic evaluation and optimization ( Fig. 1 ). Herein, the telodendrimer system provides a blueprint for the customized nanocarrier design in the delivery of a given drug. 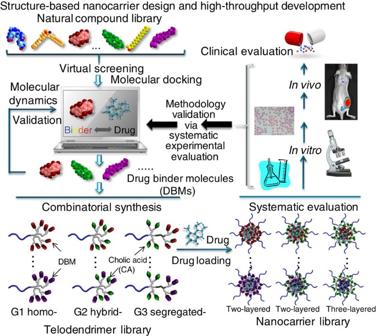Figure 1: Structure-based nanocarrier design and development. Schematic illustration of the rational design and combinatorial synthesis of telodendrimers for systematic evaluation and optimization of nanocarriers. Figure 1: Structure-based nanocarrier design and development. Schematic illustration of the rational design and combinatorial synthesis of telodendrimers for systematic evaluation and optimization of nanocarriers. Full size image Structure-based telodendrimer design To prove the concept, a number of lipophilic vitamins and natural molecules were collected into a model library for virtual screening against DOX via molecular docking. As shown in Fig. 2a , the docking energies were ranked on the basis of the mean of 100 docking assays ( Supplementary Table 1 ). DOX was not shown as the most favourable binder to itself in the docking study because of steric hindrance. As expected, the aromatic molecules, such as anthraquinone (AQ), Rhein (Rh) and 1,4-dihydroxy-2-naphthoic acid, and the polycyclic steroid molecules, for example, cholesterol (Cho), lithocholic acid (LiCA) and CA, could bind to DOX strongly with minimum docking energy of −5.65 ∼ −6.07 kcal mol −1 via pi–pi and pi -polycyclic hydrophobic interactions and hydrogen bonding, respectively. In contrast, the segments of typical synthetic polymers, for example, poly(ɛ-caprolactone) (PCL) and poly(lactic acid) and a fatty acid of heptadecanoic acid (C17) showed less negative docking energies with DOX (−0.75 ∼ −2.81 kcal mol −1 ). 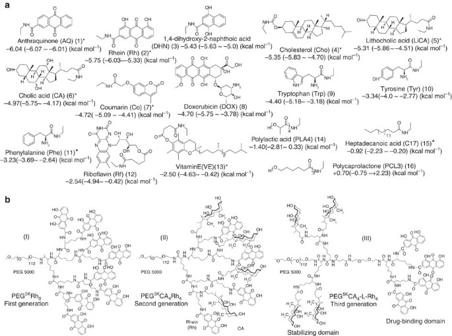Figure 2: Chemical structures of building blocks and telodendrimers. (a) Representative DBMs ranked by docking energies against DOX binding in molecular docking. The docking energies are presented as the average and the range of docking energy. *Building blocks selected for telodendrimer synthesis. (b) Three generations of telodendrimers with distinct architectures synthesized by peptide chemistry: the first generation of telodendrimers PEG5kRh8(I), second generation of telodendrimer PEG5kCA4Rh4(II) and the third generation of the functional segregated telodendrimer PEG5kCA4-L-Rh4(III). As an example, Rh is presented as one of the DBMs together with an amphiphilic CA on the periphery. Figure 2: Chemical structures of building blocks and telodendrimers. ( a ) Representative DBMs ranked by docking energies against DOX binding in molecular docking. The docking energies are presented as the average and the range of docking energy. *Building blocks selected for telodendrimer synthesis. ( b ) Three generations of telodendrimers with distinct architectures synthesized by peptide chemistry: the first generation of telodendrimers PEG 5k Rh 8 (I), second generation of telodendrimer PEG 5k CA 4 Rh 4 (II) and the third generation of the functional segregated telodendrimer PEG 5k CA 4 -L-Rh 4 (III). As an example, Rh is presented as one of the DBMs together with an amphiphilic CA on the periphery. Full size image It has been a concern that the lack of water in molecular docking decreases its accuracy in predicting binding events in an aqueous environment, for example, in the drug-loading process. To address this issue, we conducted molecular dynamic simulations on the DBM–DOX complexes in the presence of explicit water. The DBM–DOX complexes with the lowest docking energies were taken as the initial conformations for molecular dynamics (MD) simulation for 5 ns. The mean interaction energies between DBMs and DOX over the simulation were extracted ( Supplementary Table 1 ) and compared with docking energy ( Fig. 3a ). The docking energies were observed to be less negative than MD interaction energy because of the consideration of desolvation and torsion energies in Autodock 4 energy evaluation [29] . Importantly, a good monotonic correlation (Pearson’s r : 0.88) was observed for the DBMs with the relatively rigid structures, for example, aromatic or steroidal compounds with high dock rankings. However, the docking energy of flexible molecules, such as fragments of typical synthetic polymers of PCL, poly(lactic acid) and a fatty acid of C17 were underestimated by docking, which exhibited more favourable interactions in MD simulations, although still higher than those of rigid aromatic and steroidal compounds. Riboflavin (Rf) and vitamin E (VE, α-tocopherol) have both aromatic and flexible components in their structures and exhibited the most favourable interactions with DOX in MD simulation via adapting hairpin-binding models ( Supplementary Fig. 2a ). Interestingly, the binding energy for DOX-riboflavin underwent sudden changes with time, which was also observed for DOX–DOX binding ( Supplementary Fig. 2f,g ), may be due to their hydrophilic side chains. In contrast, a converging energy profile was observed for VE binding with DOX via hydrophobic interactions. 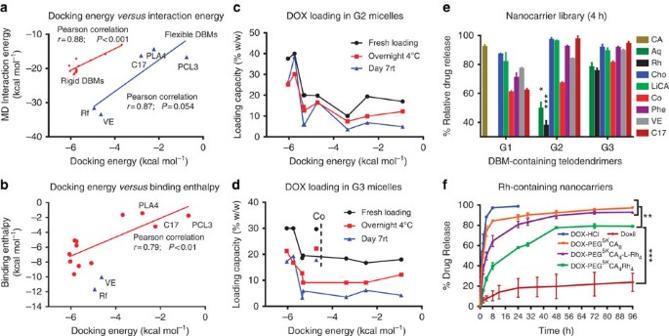Figure 3: Methodology validation and systematic evaluation. (a,b) Most favourite docking conformations between DBM and DOX were simulated by molecular dynamics for 5 ns in the presence of explicit water. (a) Unbound interaction energy computed from MD simulations plotted against the minimum docking energies. (b) The binding enthalpies analysed by a solvent-balance method were plotted against the lowest docking energies. Linear regression model was fit via Ordinary Least Square to calculate the Pearson correlation coefficient and the associatedPvalues. (c,d) Drug-loading capacities of G2 (c) and G3 (d) telodendrimer micelles at fresh loading and after storage were plotted against docking energies of the DBMs. (e) Percentage of DOX release from G1, G2 and G3 telodendrimer micelle library relative to the release rate of free DOX and PEG5kCA8at 4 h. (f)In vitrodrug release profiles were studied using a dialysis method under sink condition for free DOX, Doxil and DOX loaded in various telodendrimer nanocarriers. Data were presented as mean±s.e.m. (n=3). Student’st-test: *P<0.05; **P<0.01; ***P<0.001. Figure 3: Methodology validation and systematic evaluation. ( a , b ) Most favourite docking conformations between DBM and DOX were simulated by molecular dynamics for 5 ns in the presence of explicit water. ( a ) Unbound interaction energy computed from MD simulations plotted against the minimum docking energies. ( b ) The binding enthalpies analysed by a solvent-balance method were plotted against the lowest docking energies. Linear regression model was fit via Ordinary Least Square to calculate the Pearson correlation coefficient and the associated P values. ( c , d ) Drug-loading capacities of G2 ( c ) and G3 ( d ) telodendrimer micelles at fresh loading and after storage were plotted against docking energies of the DBMs. ( e ) Percentage of DOX release from G1, G2 and G3 telodendrimer micelle library relative to the release rate of free DOX and PEG 5k CA 8 at 4 h. ( f ) In vitro drug release profiles were studied using a dialysis method under sink condition for free DOX, Doxil and DOX loaded in various telodendrimer nanocarriers. Data were presented as mean±s.e.m. ( n =3). Student’s t -test: * P <0.05; ** P <0.01; *** P <0.001. Full size image Furthermore, the binding enthalpy of DBMs and DOX were calculated by a solvent-balance method [30] from three MD simulations for the complex, and individual molecules with the same number of water molecules before and after molecular binding ( Supplementary Fig. 3a ). The average potential energies ( U ) of the initial systems, that is, (DBM+ n H 2 O) and (DOX+ m H 2 O) and final (DBM–DOX+( m + n )H 2 O) system were analysed, as shown in Supplementary Table 2 . The enthalpy changes (Δ H ) were calculated as: It showed that the enthalpy changes were at a similar level and correlated monotonically with docking energies ( Fig. 3b ) and the MD interaction energies ( Supplementary Fig. 3c ). In addition, enthalpy calculations can differentiate the DBMs with the similar docking energies, such as aromatic molecules (Rh, AQ and 1,4-dihydroxy-2-naphthoic acid) and steroid compounds (CA, LiCA and Cho). These studies demonstrated that MD simulation provides a valuable validation for DBMs’ docking results, especially for flexible molecules. Indicated by both molecular docking and MD simulations, Rh exhibited consistent, strong DOX-binding affinities. It can be conjugated on telodendrimer through its readily available carboxylic acid functional group. In addition, Rh is an attractive bioactive molecule in traditional Chinese medicine [31] , [32] . Rh binds to DOX with much negative docking energies (−6.03 versus −4.9 kcal mol −1 ) and much narrower energy distributions (−0.76 versus 1.77 kcal mol −1 ) than DOX–DOX binding. Experimentally, 1 H NMR and nuclear Overhauser effect spectroscopy spectra of a DOX-Rh solution mixture in DMSO- d 6 indicated the correlations of both polar hydrogen and aromatic protons between DOX and Rh ( Supplementary Fig. 4a–c ), suggesting the formation of intermolecular H-bonding and pi – pi stacking. In addition, we found that DOX stabilizes Rh from crystallization in dimethyl sulfoxide (DMSO) at a concentration of ∼ 10 mM during NMR study. In contrast, only hydrogen bonding was indicated with NMR studies and no hydrophobic interactions were detected between CA and DOX in DMSO ( Supplementary Fig. 4d,e ), which correlates with a slightly higher docking energy (−5.75 kcal mol −1 ) between CA–DOX with broader energy distributions than Rh DOX (2.18 versus 0.76 kcal mol −1 ). This may be the reason for the fair stability of DOX loading in the typical CA-contacting telodendrimer PEG 5k CA 8 micelles [25] . As shown in Fig. 2b , PEG 5k Rh 8 was first prepared. It is almost insoluble in aqueous solution because of the overwhelming intermolecular pi – pi stacking and hydrogen bonding between Rh moieties. To develop an efficient nanocarrier, the strong adherent forces need to be restricted within the core of the nanocarrier for drug loading, which is achieved mostly by the PEGylation of nanoparticles. However, it is not sufficient sometimes to use the conventional PEG with chain length from 2 to 5 kDa in molecular weight to stabilize the cluster of hydrophobic components introduced in telodendrimer for optimization, such as PEG 5k Rh 8 . In our previous studies, the facial amphiphilic CA was found to be important for telodendrimers to form stable micelles, in comparison with its hydrophobic analogues [23] . We have demonstrated that the hydrophilic hydroxyl-rich surface of CA faces towards the aqueous PEG layer on the core–shell interface of PEG 5k CA 8 micelles to minimize the surface tension, therefore stabilizing the nanocarriers [33] . With this in mind, we developed another two versions of telodendrimers with the rational architecture design: that is, the second generation (G2) of hybrid telodendrimers and the third generation (G3) of functional segregated telodendrimers ( Fig. 2b ) using CA as co-building blocks. The proximal positions of CA within both G2 and G3 telodendrimers are expected to stabilize nanocarriers and payloads. As a result, G2 PEG 5k CA 4 Rh 4 and G3 PEG 5k CA 4 -L-Rh 4 were observed to be easily dispersed into aqueous solution and readily for DOX loading. Combinatorial nanocarrier synthesis and characterization In order to systematically validate the computational prediction in guiding telodendrimer design, eight representative DBMs with different docking energy levels ( Fig. 2a ) were selected for G1, G2 and G3 telodendrimer synthesis, respectively. Table 1 shows 24 telodendrimers synthesized in a combinatorial manner by conjugating DBMs on the periphery of polylysine scaffolds ( Supplementary Fig. 1 ). All the telodendrimers were fully characterized by 1 H NMR and MALDI-TOF MS ( Supplementary Fig. 10 ). As expected, most of the G1 telodendrimers have poor solubility with polydispersed particle sizes, especially for DBMs with high partition coefficient (logP), for example, Cho, LiCA, C17 and VE, which are commonly used as building blocks in amphiphilic polymer micelle preparation. Alike PEG 5k Rh 8 , an AQ-containing telodendrimer PEG 5k AQ 8 has very poor solubility in aqueous solution because of its overwhelming pi–pi stacking. In contrast, G1 telodendrimer derivatives from smaller DBMs, for example, coumarin (Co) and phenylalanine self-assemble into micelles with uniform and small particle sizes of ∼ 35 and 42 nm, respectively. In addition, these two telodendrimers exhibited relatively good DOX-loading capacities with ∼ 20–30% drug loading. G2 and G3 telodendrimers mostly formed well-dispersed micelles with sub-40 nm size before and after DOX loading at a 20% feed content with good to excellent loading efficiency. Throughout the library of the 24 nanocarriers, Rh- and AQ-containing G2 and G3 telodendrimers represent the best nanocarriers with ∼ 30 ∼ 40% (w/w) of DOX-loading capacity and ∼ 100% initial loading efficiency ( Fig. 3c,d ). Table 1 Drug-loading properties of nanocarrier library. Full size table As shown in Table 1 , critical micelle concentrations of the telodendrimer micelles in the library are mostly less than 3 μM, indicating stable micelle construction. The DOX release profiles from all micelle formulations were tested using dialysis methods. The G1 telodendrimer nanocarriers released the drug slower than G2 and G3 telodendrimers with the same building blocks, likely because of the significantly reduced drug contents after removal of drug precipitations as well as the enhanced entanglement and larger particle sizes. Of the DBMs tested, Rh- and AQ-containing G2 telodendrimers sustained DOX better from release ( Fig. 3e ) and exhibited the best stabilities ( Table 1 ) than all other formulations. In contrast, a significant amount of drug precipitations were observed on storage for all other formulations, including G1-Ph, G1-Co and G3-Co nanocarriers. Overall, the drug-loading capacity and stability of DOX-loaded telodendrimer correlated with the DOX-binding affinities of DBMs as evaluated computationally. Given the rationally designed architectures, the drug-binding affinity of a nanocarrier can be increased without sacrificing the stability and dispersibility of nanocarriers. Characterization of Rh-containing telodendrimer nanocarriers DOX release profiles from G2 and G3 Rh-containing telodendrimer micelles were then compared with free DOX, Doxil and DOX-PEG 5k CA 8 ( Fig. 3f ). As expected, a burst release and a very slow drug release of DOX were observed, respectively, for free DOX and stealth liposomal Doxil. DOX-loaded PEG 5k CA 8 formulation was observed similarly to the free DOX release profile. DOX release was significantly slower from G2 telodendrimer PEG 5k CA 4 Rh 4 than G3-Rh telodendrimer, DOX-PEG 5k CA 8 and free DOX. After DOX loading, the critical micelle concentrations of the G2-Rh and G3-Rh micelles were slightly decreased to 0.83 and 1.1 μM, respectively ( Table 1 ), using Nile Red (NR) as a fluorescent probe [34] . Interestingly, NR as well as DOX were fluorescently quenched after being loaded in Rh-containing G1 and G2 telodendrimer micelles, indicating the close pi – pi interactions between DOX or NR with Rh moieties in telodendrimers ( Supplementary Fig. 5a,b ). In contrast, the fluorescent signal of DOX was enhanced after being loaded in non-aromatic PEG 5k CA 8 micelles ( Supplementary Fig. 5e ). Meanwhile, pronounced fluorescent signals were observed after DOX or NR was loaded in the G3-Rh telodendrimer nanocarriers ( Supplementary Fig. 5c,e ). This suggests that DOX or NR can be encapsulated partially in the CA-rich proximal layer in the domain-segregated G3-Rh micelles ( Supplementary Fig. 5f ) and remain fluorescent. This also explains the relatively faster DOX release from G3-Rh micelles than that from G2-Rh micelles because of the lower DOX-CA-binding affinity. The reproducibility and quality control of nanocarrier synthesis is critical for clinical development of nanomedicine. To test the reproducibility, G2 and G3 Rh/CA-containing telodendrimers were re-synthesized following the procedure shown in Supplementary Fig. 1 . Both NMR and MALDI-TOF MS analyses revealed the precise telodendrimer synthesis via peptide chemistry ( Supplementary Fig. 6a–d ). The G2 and G3 Rh-telodendrimers self-assemble into uniform micelles with sizes of 17 and 32 nm, respectively, determined with the dynamic light scattering (DLS) analysis ( Supplementary Fig. 6e ). Transmission electron microscopy (TEM) images revealed spherical micelles formed by G2 hybrid PEG 5k CA 4 Rh 4 telodendrimer before and after DOX loading. In contrast, the G3 telodendrimers self-assemble into short rod-shaped micelles ( ∼ 10 nm in width) before and after DOX loading. Segregated oligo-Rh in the G3 telodendrimer has a good chance to form the long range pi–pi stacking in one dimension, whereas Rh is separated by CA in the G2 hybrid telodendrimer. TEM indicated the increased thickness of G3 worm-like micelles from 10 to 16 nm with increasing DOX loading contents from 10 to 30% by weight ( Supplementary Fig. 6f,g ). Proton NMR spectra of the fresh DOX-loaded micelle solutions in D 2 O were recorded with no recognizable free DOX signals detected, indicating the completion of drug encapsulation (data not shown). The DOX-loaded G2 and G3 micelle solutions at 20% drug content maintained stable particle size and drug-loading content on storage at 4 °C for months monitored using DLS and UV–vis spectroscopy, respectively, while precipitation usually appears for DOX-loaded PEG 5k CA 8 micelles at 4 °C overnight. Given the enhanced stability, the haemolytic activities of both G2 and G3 Rh-containing telodendrimers were almost undetectable before and after DOX loading up to 1 mg ml −1 concentration after 4 h and overnight incubation with red blood cells (RBCs) in vitro ( Fig. 4a ). DOX-PEG 5k CA 8 was observed to have moderate haemolysis ( ∼ 20%) at 1 mg ml −1 , despite very low haemolysis for the blank ones (<5%). Reduced drug uptake in Raji lymphoma cells was observed in the cell lysate after incubation with both G2 and G3 DOX nanoformulations when compared with free DOX and DOX-PEG 5k CA 8 ( Fig. 4b , Supplementary Fig. 7a–c ). Doxil had even lower cell uptake after 30-min incubation, reflecting the stealth property and superior drug encapsulation stability. The cell uptake of G2 and G3 telodendrimer micelles and Doxil were significantly enhanced at 37 °C when compared with that at 4 °C in a concentration-dependent manner, indicating nanoparticle uptake through the endocytosis pathway. As expected, reduced cytotoxicity of Doxil, DOX-G2-Rh and DOX-G3-Rh formulations on Raji lymphoma cells was observed after a drug exposure of 30 min ( Fig. 4c ) or 2 h ( Supplementary Fig. 7d ), which was correlated with the reduced cell uptake. This may indicate reduced off-target toxicity of payload drug in blood circulation. Blank G2-Rh and G3-Rh telodendrimer micelles did not show toxicity at a concentration of 500 μg ml −1 in cell culture. As shown in the in vitro cell viability assays after a 72-h drug incubation in three lymphoma cell lines ( Fig. 4d , Supplementary Fig. 7e–h ), the telodendrimer nanoformulations of DOX exhibited similar half-maximum growth inhibitory concentrations (IC50s) compared with free DOX because of the efficient drug release as shown in Fig. 3f . While Doxil exhibited ∼ 40- to 100-fold reduction in IC50 compared with the other formulations, which was because of reduced cell uptake ( Fig. 4b ) and slow drug release ( Fig. 3f ). It demonstrated that the balanced drug sustainability and drug release are important to reduce side effects and maximize drug efficacy. 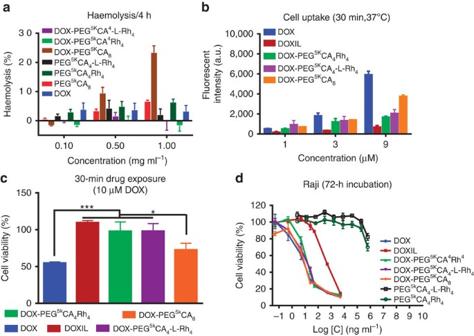Figure 4: Biocompatibility and cytotoxicity of optimized nanoformulations. (a) Reduced haemolytic properties of Rh-containing optimized telodendrimers with/without DOX loading after incubation with red blood cell at 37 °C for 4 h. (b) Slower cell uptake of optimized nanoformulations measured by the fluorescent signals of the cell lysate of Raji lymphoma cells after the incubation with free DOX, Doxil and three DOX nanoformulations with concentrations of 1, 3 and 9 μM at 37 °C for 30 min. (c) Reduced cytotoxicity of nanoformulations to Raji cells after being incubated with various DOX formulations for 30 min, followed by the incubation with refreshed cell culture medium for 72 h. (d) Maintained efficacy of optimized nanoformulations on Raji lymphoma cells after continuous 72 h incubation with blank micelles, free DOX, Doxil and DOX nanoformulations. Data were presented as mean±s.e.m. (n=3). Student’st-test: *P<0.05; **P<0.01; ***P<0.001. Figure 4: Biocompatibility and cytotoxicity of optimized nanoformulations. ( a ) Reduced haemolytic properties of Rh-containing optimized telodendrimers with/without DOX loading after incubation with red blood cell at 37 °C for 4 h. ( b ) Slower cell uptake of optimized nanoformulations measured by the fluorescent signals of the cell lysate of Raji lymphoma cells after the incubation with free DOX, Doxil and three DOX nanoformulations with concentrations of 1, 3 and 9 μM at 37 °C for 30 min. ( c ) Reduced cytotoxicity of nanoformulations to Raji cells after being incubated with various DOX formulations for 30 min, followed by the incubation with refreshed cell culture medium for 72 h. ( d ) Maintained efficacy of optimized nanoformulations on Raji lymphoma cells after continuous 72 h incubation with blank micelles, free DOX, Doxil and DOX nanoformulations. Data were presented as mean±s.e.m. ( n =3). Student’s t -test: * P <0.05; ** P <0.01; *** P <0.001. Full size image Reduced toxicity and increased tumour targeting The maximum tolerated doses (MTDs) of different DOX formulations were tested in BALB/c mice ( Supplementary Fig. 8a,b ). A single dose MTD of a G2 DOX-PEG 5k CA 4 Rh 4 was determined to be between 20 and 25 mg kg −1 , which is ∼ 2- to 2.5-fold higher than the MTD dose of DOX and Doxil (10 mg kg −1 ) [25] . The MTD for G3 of DOX-PEG 5k CA 4 -L-Rh 4 was observed to be between 15 and 20 mg kg −1 . The blank G2-Rh and G3-Rh telodendrimer micelles were tested in animals: no toxicity and no body weight loss were observed after a single injection at 125 mg kg −1 . In order to identify proper doses for in vivo cancer treatment, repeated dosages were given at a dose of 15 mg kg −1 on days 0 and 4. The G2 DOX-PEG 5k CA 4 Rh 4 nanoformulation was tolerated well in the animals. One animal receiving G3 DOX-PEG 5k CA 4 -L-Rh 4 was killed on day 9 because of body weight loss over 30%. All other animals in this treatment group had a weight loss of less than 15%. The higher toxicity of G3 formulation may be related to the faster drug release profile. The total DOX concentrations in the plasma of mice were determined by fluorescent measurements after intravenous administration of free DOX and DOX nanoformulations ( Fig. 5a ). Free DOX was eliminated rapidly from circulation. Consistent with the previous report [25] , Doxil had an extremely long circulation time with ∼ 85% and 35% of drug detected at 5 min and 24 h post injection, respectively. Similar to free DOX, only 8% of DOX-PEG 5k CA 8 was detected at 5 min, indicating its poor in vivo stability for drug encapsulation. In contrast, Rh-containing G2 and G3 telodendrimer nanocarriers showed remarkably prolonged blood circulation, with more than 63 and 54% of the injected dosage retained in blood after 5 min, and 7.3% of G2 and 7.9% of G3 were detected at 24 h post injection. A pharmacokinetics (PK) analysis using a three-compartment model was performed for both free drug and nanoformulations ( Supplementary Table 3 ). Compared with free DOX administration, Doxil has a ∼ 37-fold slower elimination constant (K01) and 36-fold increase in area under curve (AUC) of the plasma drug concentration. The stealth PEG layer and the stable crystallized DOX in Doxil enabled the extremely prolonged drug circulation. DOX-PEG 5k CA 8 was observed to have a similar PK profile with free drug, which correlates with its low drug-binding affinity and poor in vitro stability. In contrast, Rh-containing G2 and G3 nanoformulations of DOX showed significantly improved PK profiles with greater than a sixfold decrease in K01 and a sixfold increase in plasma AUC than free DOX and DOX-PEG 5k CA 8 . Similar to the reported studies [8] , Doxil had a terminal half-life ( t 1/2 ) of 32.8 h, the longest one among all the formulations. In comparison, G2 and G3 DOX nanoformulations consistently prolonged t 1/2 to ∼ 11 h, which was increased 72-fold when compared with that of free DOX. Consistently, the steady-state volume of distribution ( V ss ) of Doxil is very small, 0.076 l kg −1 , which approximates the blood volume of animal, indicating the dominant blood pool residency. Similarly, both G2 and G3 Rh-containing formulations have a small V ss of 0.12 l kg −1 . However, free DOX and DOX-PEG 5k CA 8 have about more than a 10-fold increase in V ss , 1.35 and 1.26 l kg −1 , respectively, indicative of rapid distribution/dispersion of free drug and unstable nanoformulations into the tissues in mice. 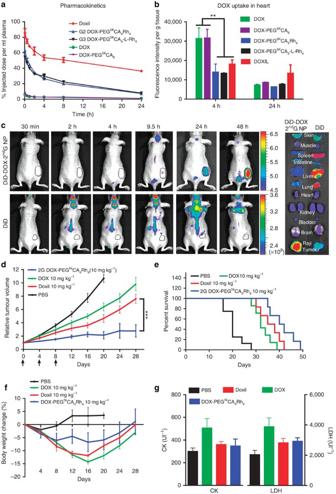Figure 5:In vivoperformance of nanoformulations. (a) PK profiles of DOX concentration in plasma and (b) drug uptake in the heart analysed at different time points after tail vein injection of free DOX, Doxil and DOX-loaded micelles at a dose of 10 mg kg−1in BALB/C mice (5–6 weeks, both sexes). (c)In vivoandex vivonear NIRF optical images of Raji lymphoma-bearing nude mice (∼10 weeks, female) injected intravenously with free DiD dye and DiD-DOX-co-loaded G2 PEG5kCA4Rh4micelles, respectively. Tumours and major organs were excised forex vivoimaging at 48 h post injection. (d)In vivotumour growth inhibition, (e) Kaplan–Meier survival curve and (f) body weight changes of Raji lymphoma-bearing nude mice (9–11 weeks, both sexes) treated with different DOX formulations at 10 mg kg−1for three doses on days 0, 4 and 8 (n=5–8) on nude mice bearing Raji lymphoma tumours with the initial volume of 100–150 mm3. (g) The serum CK and LDH levels were analysed 7 days after the last treatment. Data were presented as mean±s.e.m. Student’st-test: *P<0.05; **P<0.01; ***P<0.001. Figure 5: In vivo performance of nanoformulations. ( a ) PK profiles of DOX concentration in plasma and ( b ) drug uptake in the heart analysed at different time points after tail vein injection of free DOX, Doxil and DOX-loaded micelles at a dose of 10 mg kg −1 in BALB/C mice (5–6 weeks, both sexes). ( c ) In vivo and ex vivo near NIRF optical images of Raji lymphoma-bearing nude mice ( ∼ 10 weeks, female) injected intravenously with free DiD dye and DiD-DOX-co-loaded G2 PEG 5k CA 4 Rh 4 micelles, respectively. Tumours and major organs were excised for ex vivo imaging at 48 h post injection. ( d ) In vivo tumour growth inhibition, ( e ) Kaplan–Meier survival curve and ( f ) body weight changes of Raji lymphoma-bearing nude mice (9–11 weeks, both sexes) treated with different DOX formulations at 10 mg kg −1 for three doses on days 0, 4 and 8 ( n =5–8) on nude mice bearing Raji lymphoma tumours with the initial volume of 100–150 mm 3 . ( g ) The serum CK and LDH levels were analysed 7 days after the last treatment. Data were presented as mean±s.e.m. Student’s t -test: * P <0.05; ** P <0.01; *** P <0.001. Full size image About a 50% reduction in heart uptake of drug for Doxil and G2-Rh, G3-Rh DOX nanoformulations were observed relative to free DOX and DOX-PEG 5k CA 8 at 4 h post administrations. Despite the prolonged blood circulations, there was no significant difference in heart uptake at 24 h post injection for all formulations. The overall reduced AUC in the heart and the reduced peak values of free drug in circulation via Doxil, G2-Rh and G3-Rh DOX nanoformulations correlated with the reduced cardiotoxicity ( Fig. 5b ). The near infrared (NIR) in vivo and ex vivo imaging showed that G2-Rh DOX nanoformulation could deliver fluorescent payload to the tumour site preferentially as shown in Fig. 5c . Threefold greater tumour uptake and fourfold less uptake in the liver, lung and spleen were observed in the animals treated with G2-Rh DOX nanoformulation in comparison with the free payload administration ( Supplementary Fig. 8 ). Enhanced anticancer effects Raji lymphoma xenograft models were treated with DOX nanoformulations, free DOX and Doxil intravenously on days 0, 4 and 8 ( n =5–8) at the equivalent DOX dose of 10 mg kg −1 , which is the MTD level for free DOX and Doxil. Initial tumour volumes were 150 ∼ 200 mm 3 . As shown in Fig. 5d , DOX-G2-Rh was the most efficient one in inhibiting tumour growth ( P <0.05) with the relative tumour volume (RTV) of 2.1 on day 20. The DOX-G2-Rh treatment group also had a significantly prolonged median survival time (41 days) compared with groups treated with PBS (20 days), DOX (32 days) and Doxil (36.5 days; Fig. 5e ). The body weights of animals were monitored with a maximum loss of <15% seen in all groups, which were recovered by the week 4 ( Fig. 5f ). Similar RBC and platelet counts were observed for all the groups on day 7 after the last administration. There was slightly reduced white blood cell (WBC) numbers observed in the animals treated with free DOX ( Supplementary Table 4 ), indicating myelosupression. No liver and kidney damage was observed as indicated by stable levels of alanine amino transferase (ALT), aspartate amino transferase (AST) and blood urea nitrogen (BUN) in all groups ( Supplementary Table 5 ). Of note, the biomarkers for the cardiotoxicity, for example, serum creatine kinase (CK) and lactate dehydrogenase (LDH) were elevated significantly in animals treated with free DOX ( Fig. 5g ). G2-Rh DOX nanoformulation and Doxil did not show significant CK and LDH elevation when compared with free DOX, indicating reduced cardiotoxicity. Given the reduced toxic side effects and the increased MTD for G2-Rh and G3-Rh DOX nanoformulations, the anticancer effects could be further enhanced with higher tolerated dosages. Advanced tumours with large tumour volumes pose challenges for disease control. A separate in vivo cancer treatment study was designed to apply a higher dose (15 mg kg −1 ) of telodendrimer nanoformulations to treat animals with an average initial lymphoma tumour volume of 700 mm 3 . Two dose levels of G2-Rh and G3-Rh DOX nanoformulations, 10 and 15 mg kg −1 , were used to treat lymphoma cancers in nude mice bearing xenografted tumours for efficacy and toxicity studies. As shown in Fig. 6a , the mice tolerated three-dosage treatments of G2-Rh DOX nanoformulations at both 10 and 15 mg kg −1 with maximum body weight loss of less than 15%. All mice in the group treated with G3-Rh DOX nanoformulation died at 15 mg kg −1 after three treatments. Mice in the DOX-G3-10 mg kg −1 group survived from three dosages with maximum body weight loss less than 20% on day 14, which gradually recovered over the next 10 days. When compared with the PBS control group, none of the groups showed a decrease in the number of WBCs, RBCs, platelets or haemoglobin ( Supplementary Table 4 ). In the animals treated with G3-Rh DOX nanoformulation at 10 mg kg −1 , a slight increase in WBCs was observed (11.6±3.0 K μl −1 , normal range: 1.8–10.7). 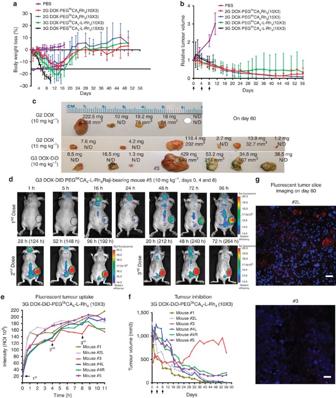Figure 6: Enhanced anticancer effects. In vivocancer treatment and theranostic tumour imaging in nude mice (9–11 weeks, both sexes) bearing Raji lymphoma tumours with the initial volume of 600–800 mm3. (a) Tumour inhibition curves and (b) body weight changes of mice after intravenous treatment with G2 and G3 nanoformulations of DOX at 10 and 15 mg kg−1, respectively, for three doses on days 0, 4 and 8 (n=5–7). PBS injection was used in the control group. (c)In vivovolume andex vivoweight of tumours in the G2 and G3 treatment groups. (d)In vivoNIRF optical images of Raji lymphoma bearing mice #5 treated with the intravenous injection of DiD–DOX-co-loaded G3 PEG5kCA4-L-Rh4micelles (10 mg kg−1) for three times on days 0, 4 and 8. (e) Fluorescent quantitative tumour uptake analysis and (f) tumour volume measurements of individual mice in the G3 DiD–DOX treatment group. (g) Lymphoma tumour tissue #2L and #3 stained with 4,6-diamidino-2-phenylindole and observed under fluorescent confocal microscope: red fluorescent is the signal from DiD and blue from nuclei. Scale bar, 20 μm. Figure 6: Enhanced anticancer effects. In vivo cancer treatment and theranostic tumour imaging in nude mice (9–11 weeks, both sexes) bearing Raji lymphoma tumours with the initial volume of 600–800 mm 3 . ( a ) Tumour inhibition curves and ( b ) body weight changes of mice after intravenous treatment with G2 and G3 nanoformulations of DOX at 10 and 15 mg kg −1 , respectively, for three doses on days 0, 4 and 8 ( n =5–7). PBS injection was used in the control group. ( c ) In vivo volume and ex vivo weight of tumours in the G2 and G3 treatment groups. ( d ) In vivo NIRF optical images of Raji lymphoma bearing mice #5 treated with the intravenous injection of DiD–DOX-co-loaded G3 PEG 5k CA 4 -L-Rh 4 micelles (10 mg kg −1 ) for three times on days 0, 4 and 8. ( e ) Fluorescent quantitative tumour uptake analysis and ( f ) tumour volume measurements of individual mice in the G3 DiD–DOX treatment group. ( g ) Lymphoma tumour tissue #2L and #3 stained with 4,6-diamidino-2-phenylindole and observed under fluorescent confocal microscope: red fluorescent is the signal from DiD and blue from nuclei. Scale bar, 20 μm. Full size image After 4 weeks, the majority of tumours shrunk dramatically in size to ∼ 30% of the initial tumour volume in all three continuous treatment groups, for example, DOX-G2-Rh at 10 and 15 mg kg −1 and DOX-G3-Rh at 10 mg kg −1 . The initial decrease was followed by the stable tumour size or further decreases to undetectable on day 60 ( Fig. 6b ). In the control group treated with PBS, tumours progressed quickly with tumour volumes over 1,500 mm 3 on day 11 post administration. The DOX-G2-Rh formulation decreased tumour size more efficiently at the elevated dose of 15 mg kg −1 . In this treatment group, four of the six tumours were not detectable by the end of treatment ( Fig. 6c ). Even 10 mg kg −1 of DOX-G2-Rh nanoformulation exhibited a superior efficacy in shrinking tumour volume until day 46, whereas one tumour recurred. The DOX-G3-Rh nanoformulation also exhibited antitumour effects in the first 3 weeks of the treatment with significant decrease in tumour volume ( Fig. 6c ). The enhanced anticancer effects of nanoformulations in large tumours might be explained by the advanced angiogenesis increasing EPR effects. To monitor tumour-targeted drug delivery, a NIR dye, DiD, was co-loaded with DOX in the G3-Rh telodendrimer micelles for the treatment group at 10 mg kg −1 . Continuous accumulation of fluorescent signals was observed on the xenografted tumours ( Fig. 6d , Supplementary Fig. 9 ). Interestingly, a unique zigzag profile of a tumour uptake in animal #3 was observed during the treatment ( Fig. 6e ). A fast efflux indicated pronounced washout effects within this tumour, which correlated with less effective treatment in animal #3 ( Fig. 6f ). A lower fluorescent signal was observed for tumour #3 on pathological studies when compared with tumor #2L ( Fig. 6g ). This demonstrated the theranostic value of the nanoformulations in combination of NIR fluorescent imaging. The replacement of NIR probe with radio isotopes will allow for the theranostic imaging in human patients via positron emission tomography or single-photon emission computed tomography techniques. Rational nanocarrier design and structural optimization are great challenges to nanocarrier-based drug delivery. It mostly relies on the empirical approaches [21] , such as compatibility/solubility analysis to predict drug loading and release properties, [35] , [36] , [37] which omit the detailed molecular interactions in drug loading. MD and Monte Carlo simulations have been applied to simulate drug-excipient interactions [38] , [39] and nanoparticle formation [40] , [41] , [42] . A computational approach to dock drug molecules into a polymer matrix provides molecular-level information on drug–matrix interaction in the random polymer aggregates [41] , [43] or dendrimer systems [44] , [45] . In fact, there is no such virtually empty pocket pre-existing in polymer aggregates for the drug molecule to diffuse in. Instead, drug loading mostly is a dynamic process of the instant co-assembly of drug–polymer complex into the core of micelle, which is too expensive for atomic molecular simulation. Overall, the capability and liability of the computational approaches in simulating polymer–drug aggregates is a bottleneck for structure-based nanocarrier design. Experimentally, combinatorial chemistry has been applied in material discovery to search for positively charged polymers [46] , [47] and lipidoids [48] for gene delivery. However, typical amphiphilic polymers have a very limited freedom and functionality for further optimization because of the monotonic nature of polymer chemistry. It is still not practical to use polymerization approaches to synthesize a large number of well-defined polymers with diverse structures for drug-loading test or for the validation of the theoretical design. In summary, significant technical difficulties lie in both theoretical nanocarrier design and precise high-throughput nanocarrier synthesis. In addition, the synergistic combination of these two approaches in nanocarrier development is still lacking [21] . The majority mass ( ∼ 75%) of the core of telodendrimer micelle is composed of DBMs on the periphery of the dendron, which has sufficient flexibility to interact with drug molecules spatially. Therefore, drug–DBM interactions determine the drug-binding affinities within nanocarrier. Such small molecular interactions between drug–DBM can be efficiently calculated and ranked through computational approaches, thus bypassing the bottleneck of computational chemistry in studying polymer aggregates. Stepwise synthetic route via peptide chemistry affords telodendrimers with well-defined and easily diversifiable chemical structures and architectures. All of these features enable the telodendrimer system to serve as a blueprint for both computational design and combinatorial synthesis of nanocarriers for systematical evaluation. The stability of a nanoformulation determines its fate and in vivo efficacy. The polymeric micelle system is a dynamic self-assembled system in nature, which dissociates on dilution and interactions with hydrophobic components in vivo . As results, some micelle formulations in clinic development have the similar PK profiles with free drug [49] , [50] , which reduces the EPR effects for tumour-targeted drug delivery. Reversible crosslinking strategies have been applied to improve the stability of nanocarriers, for example, telodendrimer micelles [27] , [51] and other delivering systems [52] for on-demand drug delivery. However, most of the crosslinking strategies are facing significant hurdles for clinical translation, such as the crosslinking efficiency, toxicity of crosslinking treatments/reagents and tedious purification process [52] . In reality, the simple system is preferred in terms of reproducibility, quality control and regulations for clinical development. As shown in this study, the stability and drug sustainability of the non-crosslinked micelles could be enhanced by engineering a nanocarrier with specific DBMs. In concept, large numbers of biocompatible molecules could be virtually screened via molecular docking to identify DBMs, which can be verified by MD simulation. MD simulation of the drug–telodendrimer interactions at the atomic level further provides hints for drug-loading properties. The resulting telodendrimer library provides numerous candidates to optimize the drug-loading capacities and stabilities for in vitro and in vivo evaluations. Targeted drug delivery by a nanoparticle formulation is based on both elongated circulation time of nanoparticle and leaky blood vessels present in solid tumours. Doxil has a superior half-life of ∼ 20–35 h in animals and 50–80 h in human adult [8] with the majority of DOX still encapsulated when detected in plasma because of the limited drug release properties of the salt form of DOX-HCl within liposomes [8] . Doxil is able to efficiently target tumours via EPR effects and can efficiently reduce the cardiotoxicity of DOX. In clinical practice, Doxil only produced a marginally improved therapeutic benefit over free DOX [53] . Owing to the large particle size of Doxil and very slow drug release, the intratumoral penetration is limited and the drug availability within tumour is reduced. Even reduced anticancer effects for cisplatin were reported after encapsulation into the stealthy lipsomes [54] . The combination of the stable drug encapsulation in the blood stream and efficient drug release at tumour sites is believed to be critical in determining the in vivo efficacy of nanotherapeutics. The smaller sizes of polymer micelles represent intrinsic merit for intratumoral drug delivery. Both G2 and G3 DOX nanoformulations exhibited a better anticancer effect than free DOX, Doxil and the less stable telodendrimer formulations [25] . This is because of the enhanced stability and prolonged blood circulation for passive tumour targeting and the smaller sizes with the steady drug release for efficient intratumoral drug delivery and cancer killing. In summary, we have demonstrated for the first time the application of molecular docking/MD simulation techniques in screening building blocks to synthesize nanocarriers for the delivery of a given drug. The computational predictions have been validated by combinatorial synthesis and systematic evaluation of a telodendrimer nanocarrier library. Rh-containing telodendrimers were identified to have the most favourable DOX-binding affinity, as well as biocompatibility and bioactivity of a building block. Novel two-layered and three-layered telodendrimers have been synthesized using amphiphilic CA as co-core forming building blocks with other DBMs, which efficiently stabilize nanocarriers into small particle sizes and prevent further aggregation. The Rh-containing G2 and G3 telodendrimer nanocarriers exhibited superior DOX-loading capacity, stability and reduced toxic side effects when compared with the typical CA-only telodendrimers. The G2 telodendrimer could sustain DOX better with a slow release profile than the G3 telodendrimer nanocarrier. The enhanced stability of the G2 and G3 nanoformulations leads to the prolonged circulation, increased MTD, reduced cardiotoxicity and enhanced tumour-targeted drug delivery. The balanced stability and drug release profiles of G2 and G3 nanoformulations yielded the significantly improved anticancer effects when compared with both free DOX and Doxil formulations. Materials and nomenclature Doxorubicin hydrochloride (DOX·HCl; Novaplus) and Doxil (Ben Venue Laboratories Inc., Bedford, OH) were obtained from the Regional Oncology Center Pharmacy, SUNY Upstate Medical University. Monomethyl-terminated poly(ethylene glycol) monoamine (MeO-PEG-NH 2 , M w 5 kDa) were purchased from JenKem Technology USA Inc. (Fmoc)lys(Boc)-OH, (Fmoc)Lys(Dde)-OH and (Fmoc)Lys(Fmoc)-OH were obtained from AnaSpec Inc. (San Jose, CA). Tetrazolium compound [3-(4,5-dimethylthiazol-2-yl)-5-(3-carboxymethoxyphenyl)-2-(4-sulfophenyl)-2H-tetrazolium, MTS] and phenazine methosulfate were purchased from Promega (Madison, WI). Rh, CA, triethylamine and all other chemicals were purchased from Sigma-Aldrich (St. Louis). The preparations of CA derivatives (CA NHS ester) were described in the previous publication [23] . A bisamino-triethylene glycol mono-succinimide linker molecule was synthesized following a reported procedure [55] . The nomenclature of the telodendrimers followed the system used in the previous publications [23] . For example, telodendrimer PEG 5k CA 8 indicates that the molecular weight of PEG is 5 kDa and there are eight CAs conjugated the periphery of polylysine; PEG 5k CA 4 Rh 4 indicates that four CAs are conjugated on the α-amino of polylysine and four Rhs are conjugated in the ɛ-amino groups of polylysine; PEG 5k CA 4 -L-Rh 4 indicates that PEG is 5 kDa and four CAs are conjugated in the intermediate layer of telodendrimer and four Rhs are conjugated in the interior layer of telodendrimer and there is a triethylene glycol linker molecule between the two layers. Molecular mechanics The three-dimensional (3D) structure of DOX and the 3D SDF files of small molecules of interest were collected from PubChem compound website and input in Meastro software package from Schodinger ( http://www.schroedinger.com ). The carboxylic acids in these molecules were pre-masked with N-ethyl amide structure to mimic the structures after conjugation in the telodendrimer. By default, MacroModel (Schrodinger) energy minimization is performed using MMFF94 force field [56] in the presence of implicit water with the normal cutoff distances in place for unbounded interactions, for example, 7 Å for van der Waals interactions and 12 Å for electrostatics and 4 Å for H-bond were applied. The minima was searched via PRCG with the maximum iterations of 2,500 and the gradient converge threshold was set as 0.05. Molecular docking The AutoDock 4 programme was used to measure docking energies between DOX and selected small molecules. The minima conformations of DOX obtained from the Macromodel were used as a receptor in docking studies. The cube size has been optimized to be 4 nm in side length. AutoDock Tools were used to add polar hydrogen and Kollman charge to receptor molecules (DOX). The number of points in x -, y - and z dimension was 60 with the spacing of 0.375 angstrom of each grid points. Lamarckian Genetic Algorithm was used. The population size was set as 150 individuals; the maximum number of evaluations was 2.5 million; the maximum number of generations was 27,000. The rate of gene mutation was set as 0.02 and the rate of crossover was 0.8. The other docking parameter options such as random number generator, energy parameters, step size parameters and output format parameters were set as default values. Over 50 small molecular candidates were docked with the DOX for 100 runs for each docking. The binding energies with the unit of kcal mol −1 were provided in the docking result. The conformations with the same binding energy are grouped in the same cluster. Molecular dynamic simulation A series of docking complexes with high to low docking energies was further examined by MD simulation with the explicit waters using the Desmond software (Desmond/Maestro academic version 2014.2) [57] , [58] and analysed using Maestro’s trajectory visualizer. The DBM–DOX complex with the lowest docking energy was input as the initial conformation for MD simulation using OPLS-2005 force field. The water box type was orthorhombic with the boundary distance of 10 Å and the water molecules were modelled with TIP3P model [59] , which was demonstrated to be a propitiate model for studying small molecular interactions [30] . No ion was added into the system. The solvated systems were relaxed with the default multistage protocol in Desmond, followed by a series of short NVT (constant number, volume and temperature) and NPT (constant number, pressure and temperature) Berendsen [60] simulations at T =10 K with varying constraints on solute and solvent atoms. MD production runs were carried out in the NPT ensemble for 10 ns for each DBM–DOX and for 5 ns for individual DBM. The temperature was regulated to 300 K with the Nose–Hoover chain thermostat [61] , [62] with a relaxation time of 1.0 ps. Pressure was regulated to 1 bar with the Martyna–Tobias–Klein barostat using isotropic coupling and a relaxation time of 2.0 ps (ref. 63 ). The RESPA integrator [64] was used to integrate equations of motions with a 2.0-fs time step for bonded and near interactions and a 6.0-fs time step for far interactions. A cutoff of 9 Å was applied to non-bonded interactions. The smooth particle mesh Ewald method [65] was used to treat long-range electrostatics with a tolerance of 10 −9 . The OPLS_2005 force field [66] , [67] was applied to the system. The interaction energies between DOX–DBMs were analysed via the ‘Simulation event analysis’ function in Desmond/Maestro, and the mean and s.d./s.e.m. of interaction energy was calculated. In addition, the average and s.d. (mean, s.d.) of total potential energies ( U ) of the DOX–DBM binding system in water, for example, U (DBM–DOX+( m+n )H2O) was calculated via ‘simulation quality analysis’ function in Desmond/Maestro using the 10-ps block length for averaging. s.e.m. was calculated based on the formula of s.e.m.=s.d./(square root of sample size). MD simulations of individual DBMs in the same condition were performed and the corresponding was analysed. A series of MD runs of DOX was performed with the increasing boundary distance from 10 to 11, 12, 13 and 15 Å to increase water molecules included in the system. It is hypothesized that the additional water molecules with the increased box boundary could be treated as bulky water because it is beyond the 9 Å cutoff for non-bounded interactions. The potential energies of the DOX–water systems were calculated and plotted against numbers of water molecules included and the standard curve was obtained with the R 2 of 1 ( Supplementary Fig. 3b ). This working plot was used to calculate the potential energy of a DOX–mH 2 O system that is required to balance water molecules ( Supplementary Fig. 3a ) in the enthalpy calculation: ΔH = − (ref. 68 ). Telodendrimer synthesis General procedure : The telodendrimers were synthesized via solution-phase peptide amide bond condensation reactions starting from MeO-PEG-NH 2 . N-terminal-protected lysine was used to synthesize the branched scaffold of telodendrimer using diisopropyl carbodimide (DIC, 3 equiv) and N-hydroxybenzotriazole (HOBt, 3 equiv) as coupling reagents in dimethylformamide (DMF). On the negative Kaiser test of the reaction, the ice-chilled ether was added to the reaction solution to precipitate polymer, which was further washed twice with chilled ether. Fmoc-protecting groups were removed by the treatment with 20% piperidine in DMF for 30 min. Polymer was precipitated and washed with chilled ether. G1 homo telodendrimer PEG 5k -DBM 8 synthesis : A dendritic polylysine was synthesized via three repeated (Fmoc)Lys(Fmoc)-OH coupling as mentioned above. At the end, the polylysine was capped with NHS ester of DBM or DBM with free acid groups using HOBT/DIC as coupling reagents. G2 hybrid telodendrimer PEG 5k -CA 4 DBM 4 synthesis : A dendritic polylysine with orthogonal protected α-(N-Fmoc) and ɛ-(N-Boc) amino groups was synthesized on MEO-PEG-NH 2 via two repeated (Fmoc)Lys(Fmoc)-OH coupling followed by a (Fmoc)Lys(Boc)-OH coupling via HOBt/DIC chemistry. Then, the Fmoc group was removed by the treatment of 20% piperidine in DMF, followed by the coupling of CA-OSu on the α-position of lysine. Then, Boc protecting groups were removed by the treatment with 50% trifluoroacetic acid (TFA) in DCM for 30 min. Then, DBM–NHS ester reacted with the ɛ position of lysine to generate hybrid telodendrimers. G3 three-layered telodendrimer PEG 5k -CA 4 -L-DBM 4 synthesis : A two-layered dendritic polylysine with Fmoc and Boc protections, respectively, was prepared on MEO-PEG-NH 2 using orthogonal protected lysine, (Fmoc)Lys(Boc)-OH, via HOBt/DIC coupling chemistry. After the removal of Fmoc groups, DBMs with free acid groups were coupled using HOBT/DIC as coupling reagents to the terminal end of interior dendritic polylysine. Then, CA NHS ester was finally coupled to the adjacent amino groups of branched polylysine after removal of the Boc group. Telodendrimers were precipitated and washed three times with cold ether, dialysed for purification as mentioned above. Drug loading and characterizations DOX was encapsulated into telodendrimer micelles by a thin-film and hydration method. DOX·HCl was stirred with three molar equivalent of triethylamine in chloroform (CHCl 3 )/methanol (MeOH; 10:1, v/v) for 30 min to neutralize HCl. The telodendrimer was added into the above solution at certain polymer–drug ratio. Solvents were evaporated to dryness and a thin film of homogeneous drug–telodendrimer mixture was casted on the flask wall, which was further dried under high vacuum for 30 min. Then, the polymer film was reconstituted in 1 ml PBS, followed by a 30-min sonication. The particle size distributions of drug-loaded micelles were characterized by DLS (Microtrac) and TEM (a JEOL JEM-2100 HR instrument). The stability of DOX-loaded micelles on storage was evaluated by monitoring the particle sizes of micelles using DLS. Cell culture and animals T-cell lymphoma cell lines (Jurkat and MOLT-4) and B-cell lymphoma cell lines (Raji and Ramos) were purchased from American Type Culture Collection (Manassas,VA, USA). All these cells were cultured in RPMI-1640 medium supplemented with 10% fetal bovine serum, 100 U ml −1 penicillin G and 100 μg ml −1 streptomycin at 37 °C using a humidified 5% CO 2 incubator. Specific-pathogen free BALB/c mice, both sexes, aged 5–6 weeks, were purchased from Charles River (Hollister, CA); athymic nude mice (Nu/Nu strain), both sexes, aged 6–8 weekswere purchased from Harlan (Livermore, CA). All animals were kept under pathogen-free conditions according to the AAALAC (Association for Assessment and Accreditation of Laboratory Animal Care) guidelines and were allowed to acclimatize for at least 4 days before any experiments. All animal experiments were performed in compliance with the institutional guidelines and according to the protocol approved by the Committee for the Humane Use of Animals of State University of New York Upstate Medical University. MTS assay MTS assay was used to evaluate the effects of DOX-loaded micellar NPs on the cell viability against both T- and B-lymphoma cell lines. MOLT-4, Jurkat, Raji and Ramos cells were seeded in a 96-well plate at the cell densities of 8 × 10 3 cells per well. After overnight incubation, the cells were treated with different concentrations of DOX·HCl, Doxil and DOX-loaded micelles, as well as the equivalent dose of blank micelles. After 72 h incubation, CellTiter 96 Aqueous Cell Proliferation Reagent, which is composed of MTS and an electron-coupling reagent phenazine methosulfate, was added to each well according to the manufacturer’s instructions. The cell viability was determined by measuring the absorbance at 490 nm using a microplate reader (BioTek Synergy 2). Untreated cells served as a control. Results were shown as the average cell viability of triplicate wells via a formula of [(OD treat −OD blank )/(OD control −OD blank ) × 100%]. Trypan blue staining Cytotoxicity can also be measured using trypan blue staining. Raji lymphoma cells were seeded in a 96-well plate at the cell densities of 8 × 10 3 cells per well. In addition, the cells were treated with different concentrations of DOX·HCl, Doxil and DOX-loaded micelles, as well as the untreated cells as controls. After 72-h incubation, the cell suspension was mixed with 0.4% trypan blue solution at a 1:1 v/v ratio. After 1–2 min incubation, the hemocytometer chamber was carefully and continuously filled, cells were counted under the microscope in four 1 × 1 mm squares of one chamber and the average number of live (viable, unstained) and dead (blue) cells per square were determined. The average cell viability of triplicate wells via a formula of number of viable cells counted/total tells counted (viable and dead) × 100=% viable cells. Cell lysis and drug extraction It may not be accurate to quantify cellular uptake of Doxil using flow cytometry directly because the fluorescence of DOX is quenched within the intact Doxil lipsome even after cell uptake. Therefore, we employ a cell lysis and drug extraction method to analyse quantitative cellular uptake of free DOX, Doxil and DOX nanoformulations. Briefly, 1 × 10 5 Raji cells were incubated with free DOX, Doxil and DOX-loaded micelles at different DOX concentrations (1, 3 and 9 μM) for 30 min or 2 h at 4 or 37 °C, respectively. The cells were washed with PBS three times. Then, 100 μl of extraction buffer (10% Triton X-100, deionized water and acidified isopropanol (0.75 N HCl) at a 1:2:15 volumetric ratio) were added to cells, and DOX was extracted overnight at −20 °C. The fluorescence of the supernatant was determined at excitation/emission of 470/590 nm using microplate reader (BioTek Synergy 2). Haemolysis assays One millilitre of fresh blood was collected from a BALB/c mouse by cardiac puncture under deep anaesthesia into 10 ml of PBS solution in the presence of 20 mM EDTA. RBCs were then separated by centrifugation at 1,000 g for 10 min. The RBCs were washed three times with 10 ml of PBS and re-suspended in 20 ml PBS. Diluted RBC suspension (200 μl) was incubated with polymers at a series of concentrations (100, 500 and 1000 μg ml −1 ) by gently shaking at 37 °C for 0.5 and 4 h and overnight, respectively. Free DOX was also tested at the same DOX concentration levels with the DOX-loaded nanoformulations, for example, 10, 50 and 100 μg DOX ml −1 . The cell suspension was centrifuged at 1,000 g for 5 min. The free of haemoglobin in the supernatant was determined by measuring the absorbance at 540 nm using a ultraviolet–vis spectrometer. Incubations of RBCs with Triton-100 (2%) and PBS were used as the positive and negative controls, respectively. The percent haemolysis of RBCs was calculated using the following formula: RBC haemolysis=100% × (OD sample −OD PBS )/(OD triton −OD PBS ). MTD studies Healthy specific pathogen-free BALB/c mice (5–6 weeks, both sexes) were administered intravenously with DOX·HCl, DOX-PEG 5k CA 4 Rh 4 and DOX-PEG 5k CA 4 -L-Rh 4 (5 mg ml −1 DOX in 20 mg ml −1 telodendrimer) at the dose of 5, 10, 15 and 20 mg DOX per kg body weight, respectively ( n =4−5). Mouse survival and body weight change were monitored daily for 2 weeks. At 1 week after the last injection, the blood was collected from each mouse to measure blood cell counts. The MTD was defined as the allowance of a median body weight loss of 15% and causes neither death due to toxic effects nor remarkable changes in the general signs within 2 weeks after administration. Pharmacokinetic and biodistribution analysis Healthy specific pathogen-free BALB/c mice (5–6 weeks, both sexes) were administered intravenously with DOX·HCl, Doxil, DOX-PEG 5k CA 8 , DOX-PEG 5k CA 4 Rh 4 and DOX-PEG 5k CA 4 -L-Rh 4 (2 mg ml −1 DOX in 20 mg ml −1 telodendrimer) at the dose of 10 mg DOX per kg body weight, respectively ( n =3). At different time points, for example, 5 and 30 min and 1, 2, 4, 8, 24 and 32 h post injection, 20 μl of blood samples were obtained by nicking the lateral tail vein using a sterile scalpel blade, respectively. Plasma was collected and diluted to 10-fold with DMSO for fluorescent measurements using a BioTek plate reader. After the last blood collection, mice were killed and vital organs, for example, the heart, liver, lung, spleen and kidney, were collected and homogenized and extracted with extraction buffer (triton-100/water/acidified isopropanol with 0.05 N HCl 1:2.5:15 in volume) for fluorescence detection. The pharmacokinetic parameters were calculated using a three-compartment model with PKsolver, an add-in programme in Microsoft Excel [69] . The following parameters were determined: AUC (0 to infinity), maximum drug concentration ( C max ), total body clearance (Cl), terminal half-life of DOX ( t 1/2 ), steady-state volume of distribution ( V ss ), the apparent terminal elimination rate constant ( Λ ) and the mean residence time. Fluorescence animal imaging Nude mice with subcutaneous lymphoma tumours of ∼ 8–10 mm in diameter were subjected to in vivo near infrared dye (NIRF) optical imaging. Lymphoma xenograft mouse models were established by subcutaneously injecting 1 × 10 7 Raji lymphoma cells in 100 μl of mixture of PBS and Matrigel (1:1 v/v) at the right flank in female nude mice (6–8 weeks). A hydrophobic NIRF dye (DiD) was encapsulated together with DOX into the micelles using the same method as described above. The DiD–DOX-co-loaded micelle formulation was filtered with a 0.22-μm filter to sterilize the sample. The Raji lymphoma tumour xenografts bearing nude mice were injected with free DiD and DiD–DOX-co-loaded micelles at 0.2:1:10 w/w/w ratio via the tail vein, respectively. Then, the mice were anaesthetized and optically imaged using an IVIS 200 (PerkinElmer) with the excitation at 625 nm and emission at 700 nm, at different time points (0.5, 1, 2, 4, 8, 24, 48 and 72 h). At the end of the experiment, the animals were killed, and all the major organs and tumour were excised for ex vivo imaging. The associated fluorescence intensities were determined with the Living Image software (Caliper Life Sciences) using operator-defined region of interest measurements. Confocal fluorescence microscopic imaging For the histological evaluation, the harvested tumours were frozen in O.C.T. (cryo-embedding medium) at 80 °C. The corresponding slices (10 μm) were then prepared on a Minotomecryostat, air-dried for 30 min and fixed with 4% paraformaldehyde for 10 min. The nuclei were stained with 4,6-diamidino-2-phenylindole, and the slides were mounted with cover slips and imaged with Nikon laser scanning confocal fluorescence microscopy. In vivo antitumour efficacy studies Subcutaneous Raji lymphoma xenograft mouse models were used to evaluate the therapeutic efficacy of different formulations of DOX. Lymphoma xenograft mouse models were established by subcutaneously injecting 1 × 10 7 Raji lymphoma cells in 100 μl of mixture of PBS and Matrigel (1:1 v/v) at the right flank of nude mice (6–8 weeks of both sexes). When tumour volume reached 150–300 mm 3 , mice were intravenously administrated with PBS, DOX·HCl, Doxil, DOX-PEG 5k -CA 4 Rh 4 at the dose of 10 mg kg −1 DOX equivalent (MTD of free DOX), respectively ( n =5–8). In an alternative efficacy study, average tumour volume reached to ∼ 500 mm 3 before treatment to evaluate the effects of the angiogenesis. The treatments were given every 4 days on days 0, 4 and 8 for overall three doses. Tumour sizes were measured with a digital caliper twice per week. Tumour volume was calculated by the formula ( L × W 2 )/2, where L is the longest and W is the shortest in tumour diameters (mm). To compare between groups, relative tumour volume was calculated at each measurement time point (where RTV equals the tumour volume at a given time point divided by the tumour volume before initial treatment). For humane reasons, animals were killed when the implanted tumour volume reached 2,000 mm 3 , which was considered as the end point of survival data. On day 7 after the last dosage, blood samples were obtained from all the mice for the measurement of blood cell counts, hepatic or renal function tests (ALT, AST and BUN), and serum enzyme markers of cardiotoxicity including CK and LDH. One mouse from each group was also killed, and its heart was submitted for histopathology evaluation. Statistical analysis Data are presented as means±s.e.m. Linear regression model was fit via ordinary least square in the correlation studies. The Pearson correlation coefficient and the associated P values were calculated to examine the correlation between molecular bindings obtained from molecular docking and molecular simulation. Cell viability curves were fit by a three-parameter model including top, bottom and IC50. The difference ( P values) of IC50 between groups was tested by Wald z -test using the s.e. from the curve fitting. The level of significance in all statistical analyses was set at a probability of P <0.05. Statistical analysis was performed by Student’s t -test for comparison of two groups with specific variations, and one-way analysis of variance for multiple groups, followed by Newman–Keuls test if overall P <0.05. How to cite this article: Shi, C. et al. A drug-specific nanocarrier design for efficient anticancer therapy. Nat. Commun. 6:7449 doi: 10.1038/ncomms8449 (2015).